Integrated photonic quantum gates for polarization qubits The ability to manipulate quantum states of light by integrated devices may open new perspectives both for fundamental tests of quantum mechanics and for novel technological applications. However, the technology for handling polarization-encoded qubits, the most commonly adopted approach, is still missing in quantum optical circuits. Here we demonstrate the first integrated photonic controlled-NOT (CNOT) gate for polarization-encoded qubits. This result has been enabled by the integration, based on femtosecond laser waveguide writing, of partially polarizing beam splitters on a glass chip. We characterize the logical truth table of the quantum gate demonstrating its high fidelity to the expected one. In addition, we show the ability of this gate to transform separable states into entangled ones and vice versa. Finally, the full accessibility of our device is exploited to carry out a complete characterization of the CNOT gate through a quantum process tomography. Incorporating the laws of quantum mechanics in data storage, processing and transmission may unleash new possibilities for information processing, ranging from quantum communication to quantum sensing, metrology, simulation and computing [1] , [2] , [3] , [4] . In the last few years photonic quantum technologies have been adopted as a promising experimental platform for quantum information science [3] . The realization of complex optical schemes consisting of many elements requires the introduction of waveguide technology to achieve desired scalability, stability and miniaturization of the device. Recently, silica waveguide circuits on silicon chips have been employed in quantum applications to realize stable interferometers for two-qubit entangling gates [5] . Such approach with qubits encoded into two photon optical paths, representing the logical basis {|0〉,|1〉}, yielded the first demonstration of an integrated linear optical controlled-NOT (CNOT) gate. In addition, quantum walk on a chip [6] , [7] and enhanced quantum sensitivity in phase-controlled interferometers have been demonstrated with the same technology [8] , [9] , [10] , [11] . However, many quantum information processes and sources of entangled photon states are based on the polarization degree of freedom [4] , [12] , which allows one to implement quantum operations without the need of path duplication and thus with the simplest and most compact circuit layout. Up to now, integrated devices able to efficiently guide and manipulate polarization-encoded photonic qubits are still lacking [13] . Femtosecond laser waveguide writing has been emerging as a powerful tool in the rapidly advancing field of quantum photonics [14] . This technique, which was first introduced by Davis et al . in 1996 (ref. 15 ), exploits nonlinear absorption of focused femtosecond pulses to induce permanent and localized refractive index increase in transparent materials. Waveguides are directly fabricated in the bulk of the substrate by translation of the sample at constant velocity with respect to the laser beam, along the desired path. This maskless and single-step technique allows fast and cost-effective prototyping of new devices, potentially exploiting also three-dimensional geometries impossible to obtain with conventional lithography. Several devices, from simple Y-splitters [16] to increasingly complex ones [17] , [18] , [19] , have been demonstrated with applications ranging from telecommunications to integrated biosensing [20] , [21] . This technique is capable of producing high-quality waveguides with low birefringence, which are indeed suited for the propagation of polarization-encoded qubits, as we recently reported in refs 22 , 23 , where a polarization-insensitive directional coupler has been demonstrated. Here we report on the first integrated photonic CNOT gate for polarization-encoded qubits and on the complete characterization of its quantum behaviour. The demonstration of this quantum gate has been made possible by the fabrication in a glass chip of integrated devices acting as partially polarizing beam splitters (PPBSs). Precisely, we show that femtosecond laser writing enables direct inscription of directional couplers with fine and independent control on the splitting ratio for the horizontal (H) and vertical (V) polarizations. Directional couplers as partially polarizing beam splitters Directional couplers are the integrated optical analogue of bulk beam splitters (BSs) and are thus fundamental building blocks of quantum optical circuits. In these devices (see the schematic representation in Fig. 1a ) two distinct waveguides are brought close together for a certain propagation length, called interaction length, so that the two propagating modes become coupled through evanescent field overlap. In analogy to bulk BSs, reflectivity and transmissivity ratios of the directional coupler can be conveniently defined: when light is launched into port IN1 ( Fig. 1a ), R=P OUT1 /( P OUT1 + P OUT2 ) and T =1− R = P OUT2 /( P OUT1 + P OUT2 ), respectively ( P indicates the optical power); the symmetry of the device guarantees that the same relations hold when light is launched into port IN2, by simply inverting the two indices. Optical power transfer from one waveguide to the other follows a sinusoidal law with the interaction length, whose oscillation period (beating period) depends upon the coupling coefficient of the two guided modes according to coupled mode theory [24] . If some waveguide birefringence is present, the coupling coefficient, and hence the beating period, can be different for the two polarizations ( Fig. 1b ). With high birefringence waveguides, this aspect has been exploited to implement polarizing beam splitters for telecom applications [25] . 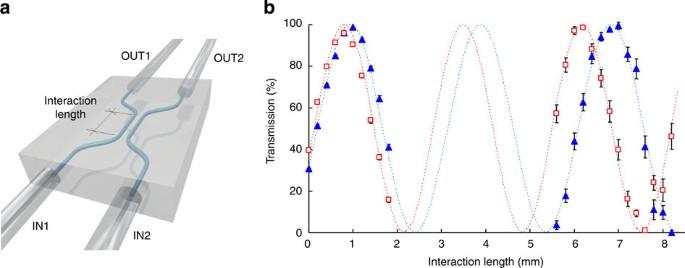Figure 1: Partially polarizing directional couplers. (a) Schematic representation of a waveguide directional coupler; IN1 and IN2 are the input ports, whereas OUT1 and OUT2 are the output ports of the device. (b) H (squares) and V (triangles) polarization transmissions of directional couplers with different interaction lengths, based on slightly birefringent waveguides. First, the 0–2 mm interaction length range was investigated to evaluate the beating length difference between the two polarizations; the interval of interest to obtain the required PPDCs was estimated to be in the 5.6–8.2 mm range, which was consequently explored. Transmission for 0 mm interaction length is non-zero, because some coupling already occurs in the curved portions of the approaching/departing waveguides. Error bars indicate fabrication reproducibility. Figure 1: Partially polarizing directional couplers. ( a ) Schematic representation of a waveguide directional coupler; IN1 and IN2 are the input ports, whereas OUT1 and OUT2 are the output ports of the device. ( b ) H (squares) and V (triangles) polarization transmissions of directional couplers with different interaction lengths, based on slightly birefringent waveguides. First, the 0–2 mm interaction length range was investigated to evaluate the beating length difference between the two polarizations; the interval of interest to obtain the required PPDCs was estimated to be in the 5.6–8.2 mm range, which was consequently explored. Transmission for 0 mm interaction length is non-zero, because some coupling already occurs in the curved portions of the approaching/departing waveguides. Error bars indicate fabrication reproducibility. Full size image However, high birefringence waveguides are not suitable for the propagation of polarization-encoded qubits as they would cause decoherence between the photons typically generated by parametric down conversion, which are characterized by a large bandwidth Δλ>1 nm. The optimal waveguides for a polarization-based quantum gate would therefore need to find the best compromise on the birefringence value, which should be low enough to preserve the coherence between photons, and high enough to enable polarization-dependent processing. Such compromise is found in femtosecond laser written waveguides in a borosilicate glass. In fact, thanks to their low birefringence, these waveguides allow to propagate polarization-encoded qubits without any perturbation and also to achieve practically polarization-insensitive devices, as demonstrated in refs 22 , 23 . However, in this work we demonstrate that the same waveguides are also capable of performing polarization-based processing of the qubits. In fact, if sufficiently long interaction lengths, covering a few beating periods, are implemented in directional couplers, it is possible to strongly enhance the difference in the polarization behaviour of the device. This approach, as shown in Figure 1b , allows to finely tailor the splitting ratios for the two polarizations and enables us to realize integrated PPBSs for the first time. Integrated quantum gates for polarization-encoded qubits We will now demonstrate how this technology can be exploited to realize quantum optical gates. In the polarization-encoding approach, a generic qubit α|0〉+β+1〉 is implemented by a coherent superposition of H and V polarization states, α| H 〉+β| V 〉, of single photons. To achieve universal quantum computation, single qubit transformations together with a two-qubit gate are sufficient [26] . One-qubit logic gates are straightforwardly implemented by using birefringent waveplates. The most commonly exploited two-qubit gate is the CNOT that flips the target qubit (T) depending on the state of the control one (C). The CNOT action is described by a unitary transformation acting on a generic superposition of two qubit quantum states. In the computational basis {|00〉,|01〉,|10〉,|11〉} for the systems C and T, the matrix associated to the CNOT is: A striking feature of this gate is given by the ability to entangle and disentangle qubits. Precisely, the input states |±〉 C |0〉 T and |±〉 C |1〉 T , where , evolve into the following output states and , which are the so-called Bell states. Photonic two-qubit gates need an interaction between the two photons that carry the information, and this would suggest that a strong optical nonlinearity is required. However, it was demonstrated that scalable quantum computing is possible by using only linear optical circuits, mainly consisting of beam splitters [28] . The most simple scheme to implement the polarization CNOT exploits three PPBSs with suitable polarization-dependent transmissivites [29] , [30] . The two-photon interaction occurs by a Hong–Ou–Mandel effect [31] in a single PPBS, whereas the other two PPBSs operate as compensators. Up to now such a scheme has been experimentally implemented only using bulk optics [32] , [33] , [34] , [35] or fibre couplers [36] . 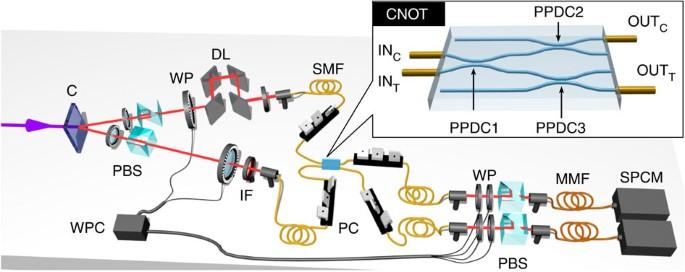Figure 2: Experimental setup. Sketch of the experimental setup that can be conceptually divided into three parts. The first part is the source: photon pairs at wavelength λ=806 nm are generated via spontaneous parametric down conversion in a 1.5 mm β-barium borate crystal (C) cut for type-II non-collinear phase matching, pumped by a CW diode laser with powerP=50 mW (ref.27). Photon polarization states are prepared by using polarizing beam splitters (PBSs) and waveplates (WPs). A delay line (DL) is inserted to control the temporal superposition of the photons, which are then coupled to single mode fibres (SMFs) and injected into the integrated CNOT gate. Interference filters (IFs) determine the photon bandwidth Δλ=6 nm. The second part shows the integrated CNOT for polarization-encoded qubits (see inset) realized by ultrafast laser writing technique. The final part represents the analysis apparatus: the polarization state of qubits emerging from the chip is analyzed by standard analysis setups (WP+PBS). Photons are then delivered to single photon counting modules (SPCM) through multimode fibres (MMFs) and coincidences between the two channels are measured. Polarization controllers (PCs) are used before and after the CNOT device to compensate polarization rotations induced by the fibres. A waveplate controller (WPC) drives the motorized waveplates to automatize the measurements. The integrated CNOT gate is achieved by the optical scheme given in the inset of Figure 2 : it consists of a first partially polarizing directional coupler (PPDC1), with transmissivities T H (1) =0 and for horizontal and vertical polarization, respectively, where target and control qubits interfere, followed by two other directional couplers (PPDC2 and PPDC3), with and , where the horizontal and vertical polarization contributions are balanced. In this scheme, the following correspondence between logical qubits and physical states holds: |0〉 C ≡| V 〉 C , |1〉 C ≡| H 〉 C , |0〉 T ≡| A 〉 T , |1〉 T ≡| D 〉 T where and . The CNOT operation succeeds with probability . Figure 2: Experimental setup. Sketch of the experimental setup that can be conceptually divided into three parts. The first part is the source: photon pairs at wavelength λ=806 nm are generated via spontaneous parametric down conversion in a 1.5 mm β-barium borate crystal (C) cut for type-II non-collinear phase matching, pumped by a CW diode laser with power P =50 mW (ref. 27 ). Photon polarization states are prepared by using polarizing beam splitters (PBSs) and waveplates (WPs). A delay line (DL) is inserted to control the temporal superposition of the photons, which are then coupled to single mode fibres (SMFs) and injected into the integrated CNOT gate. Interference filters (IFs) determine the photon bandwidth Δλ=6 nm. The second part shows the integrated CNOT for polarization-encoded qubits (see inset) realized by ultrafast laser writing technique. The final part represents the analysis apparatus: the polarization state of qubits emerging from the chip is analyzed by standard analysis setups (WP+PBS). Photons are then delivered to single photon counting modules (SPCM) through multimode fibres (MMFs) and coincidences between the two channels are measured. Polarization controllers (PCs) are used before and after the CNOT device to compensate polarization rotations induced by the fibres. A waveplate controller (WPC) drives the motorized waveplates to automatize the measurements. Full size image The PPDCs have been fabricated by the femtosecond laser waveguide writing technique above described. To calibrate the fabrication parameters, several directional couplers have been produced with different interaction lengths ranging from 0 mm to 2 mm and from 5.6 mm to 8.2 mm (see Fig. 1 ). The distance between the two waveguides in the interaction region was kept constant at 7 μm. It can be observed that for an interaction length L 1 ≃ 7.4 mm a device with T H =0 and is obtained, fulfilling the requirements for PPDC1, whereas a length L 2 ≃ 7 mm provides and T V =1 and can be adopted for PPDC2 and PPDC3. Several CNOTs have been fabricated according to the schematic of Figure 2 (inset) with slightly different interaction lengths around the values of L 1 and L 2 to take into account possible fabrication imperfections. The footprint of each integrated CNOT is 500 μm×3 cm. After characterization with a classical laser source, the devices providing the best estimated performance have been selected. The device used in the experiments has the following parameters: , , , , , and . To improve the robustness and stability of the device, single-mode fibre arrays have been permanently bonded to the input and output ports. Quantum measurements As a first quantum experiment we determined the truth table of the device operated as a CNOT gate. On this purpose we used the experimental setup represented in Figure 2 . Temporal superposition of photon wavepackets in PPDC1 was obtained by acting on the delay line. Then we injected into the chip the four computational basis states |0〉 C |0〉 T , |0〉 C |1〉 T , |1〉 C |0〉 T and |1〉 C |1〉 T and measured the probability of detecting each of them at the output. 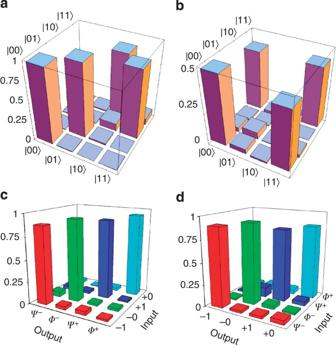Figure 3: Truth table and entanglement generation. (a) Measured truth table. (b) Experimental tomographic reconstruction of the Bell state |Φ+〉 obtained by injecting the separable state |+0〉 in the CNOT. (c) Measured probabilities of the output Bell states corresponding to the different input separable states. (d) Measured probabilities of the output separable states corresponding to the different input Bell states. The obtained truth table is reported in Figure 3a . The average measured fidelity of the logical basis [32] has been calculated as F=0.940±0.004. We can compare this value with the expected fidelity of the device , estimated by taking into account the measured transmissivities of the PPDCs. We attribute the discrepancy between the experimental and expected fidelities mainly to a partial distinguishability of photon wavepackets and non-perfect compensation of the rotation of the polarization in the single-mode optical fibres. Figure 3: Truth table and entanglement generation. ( a ) Measured truth table. ( b ) Experimental tomographic reconstruction of the Bell state |Φ + 〉 obtained by injecting the separable state |+0〉 in the CNOT. ( c ) Measured probabilities of the output Bell states corresponding to the different input separable states. ( d ) Measured probabilities of the output separable states corresponding to the different input Bell states. Full size image As already mentioned, the CNOT can also be exploited as an entangling gate. We experimentally verified this behaviour by injecting into the device the states {|±〉 C |0〉 T ,|± C |1〉 T } and measuring a set of observables to obtain a tomographic reconstruction of the density matrices of the output states. As expected the action of the CNOT converts the separable states into the maximally entangled Bell states. We report in Figure 3b one of the reconstructed density matrices and in Figure 3c the probabilities to generate the different Bell states. The fidelities of the output density matrices compared with those of the corresponding Bell states are with average value . We also checked that the CNOT gate can be adopted to discriminate the four Bell states. Indeed, the four entangled states are transformed into four orthogonal separable states, which can be easily discriminated, as shown in Figure 3d . The discrimination probability is 0.877±0.007, slightly lower than the previous fidelities due to imperfections in the entanglement source. To provide a full characterization of the quantum device we carried out a quantum process tomography [37] , first experimentally demonstrated for a CNOT gate in ref. 38 . This requires preparing the photons in a complete set of input basis states, and characterizing the output. A generic quantum process acting on a two-qubit density matrix ρ, can be expressed as where the operators Γ m are defined as tensor products of Pauli matrices {Γ m ≡σ i σ j }, i , j =0, ..., 3, m =0, ..., 15. The matrix χ mn contains all the information of the process. 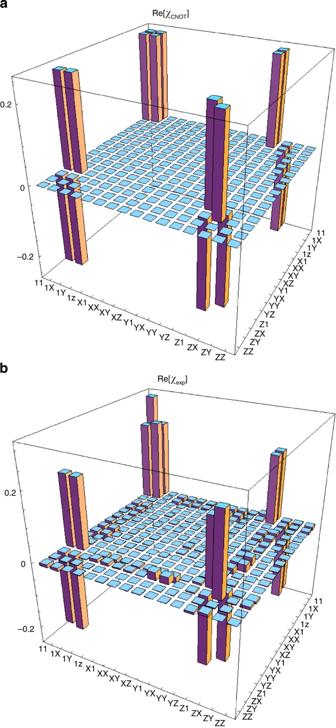Figure 4: Process matrix measurement. (a) Ideal χCNOTand (b) experimental χexpmatrices (real part) obtained from the quantum process tomography of the CNOT gate. Imaginary part of χexpis negligible.X,YandZcorrespond to Pauli matrices σ1, σ2and σ3, respectively. We reconstructed the 16×16 matrix χ exp shown in Figure 4 . The process fidelity [39] (see Methods) with the ideal CNOT gate was measured as exp =0.906±0.003. Figure 4: Process matrix measurement. ( a ) Ideal χ CNOT and ( b ) experimental χ exp matrices (real part) obtained from the quantum process tomography of the CNOT gate. Imaginary part of χ exp is negligible. X , Y and Z correspond to Pauli matrices σ 1 , σ 2 and σ 3 , respectively. Full size image We reported on the integration of partially polarizing beam splitters on a glass chip, enabling the demonstration of the first integrated photonic CNOT gate based on polarization encoding. From the fabrication point of view this work shows the capability of femtosecond laser microfabrication to produce also polarization-sensitive waveguide devices, thus further enriching the portfolio of applications that can be addressed by this simple and flexible fabrication technique. It is important to note that the polarization sensitivity/insensitivity of the directional coupler can be selected by acting on geometrical parameters and not on physical properties of the waveguides [22] , [23] . This enables simple and flexible designs of complex integrated quantum devices, where polarization-sensitive and polarization-insensitive processing can be easily cascaded. This work represents a major step towards the development of integrated photonic technology, which could provide a viable solution for quantum information processing and paves the way to the integration of a wealth of polarization-based quantum algorithms. Future research will be devoted to the on-chip implementation of both preoriented and tunable waveplates to integrate also one-qubit gates. The present results open new perspectives towards joint integrated handling of hybrid quantum states based on different degrees of freedom of light [40] , [41] , [42] , [43] , [44] , [45] , such as polarization, path and orbital angular momentum. This would significantly improve the computational power of a quantum device. The capability to process polarization-entangled photons could also benefit the quantum simulation field. As an example, exploiting the different statistics of singlet and triplet polarization-entangled states, it is possible to simulate how symmetric and antisymmetric particles travel through a quantum walk [7] , [23] , paving the way to advanced investigations on complexity physics phenomena. Chip fabrication and characterization Waveguides were micromachined in borosilicate glass substrate (Corning EAGLE2000, Corning Inc) using a commercial HighQLaser FemtoREGEN femtosecond laser, which provides 400 fs pulses at 960 kHz repetition rate. For the waveguide fabrication pulses with 240 nJ energy were focused 170 μm under the glass surface, using a 0.6 numerical aperture microscope objective whereas the sample was translated at a constant speed of 20 mm s −1 by high precision, three-axis air-bearing stages (Aerotech FiberGlide 3D, Aerotech Inc). The guided mode at 806 nm is slightly elliptical, measuring 8 μm×9 μm. Measured propagation losses are 0.8 dB cm −1 and coupling losses to single mode fibres about 1.3 dB per facet. Birefringence of these waveguides is on the order of B=7×10 −5 , as characterized in ref. 22 . For the curved segments in the directional couplers composing the integrated CNOT a 30 mm bending radius was adopted, which gives <1 dB of additional bending losses on the whole device. Quantum process tomography The full characterization of a quantum device is provided by quantum process tomography [37] . Following the procedure adopted in ref. 39 . we performed the quantum process tomography of our device and reconstructed the associated χ matrix. The experimental setup is the same one adopted in the previous measurements (see Fig. 2 ): we prepared 16 different input states and measured the projections of the output states on the set {| ij 〉}, where i , j = H , V , D , A , R , L , that is, horizontal, vertical, diagonal, antidiagonal, righthanded and lefthanded polarization, using standard polarization analysis setups. The obtained χ matrix is reported in Figure 4 . To evaluate the quality of the acquired data we calculated the process fidelity [39] as where χ CNOT is the process matrix of the ideal CNOT gate. How to cite this article: Crespi, A. et al . Integrated photonic quantum gates for polarization qubits. Nat. Commun. 2:566 doi: 10.1038/ncomms1570 (2011).